IP6K structure and the molecular determinants of catalytic specificity in an inositol phosphate kinase family Inositol trisphosphate kinases (IP3Ks) and inositol hexakisphosphate kinases (IP6Ks) each regulate specialized signalling activities by phosphorylating either InsP 3 or InsP 6 respectively. The molecular basis for these different kinase activities can be illuminated by a structural description of IP6K. Here we describe the crystal structure of an Entamoeba histolytica hybrid IP6K/IP3K, an enzymatic parallel to a ‘living fossil’. Through molecular modelling and mutagenesis, we extrapolated our findings to human IP6K2, which retains vestigial IP3K activity. Two structural elements, an α-helical pair and a rare, two-turn 3 10 helix, together forge a substrate-binding pocket with an open clamshell geometry. InsP 6 forms substantial contacts with both structural elements. Relative to InsP 6 , enzyme-bound InsP 3 rotates 55° closer to the α-helices, which provide most of the protein’s interactions with InsP 3 . These data reveal the molecular determinants of IP6K activity, and suggest an unusual evolutionary trajectory for a primordial kinase that could have favored efficient bifunctionality, before propagation of separate IP3Ks and IP6Ks. Phosphate is a universal device for imposing specificity in cell signalling. The phosphate group’s very bulk establishes geometric constraints on ligand–protein and protein–protein interactions. In addition, the phosphate’s negative charge at physiological pH bestows specificity through ionic and hydrogen bonding to only certain amino-acid residues. Signalling specificity is further enhanced through interactions that utilize multiple phosphates, such as those that are placed in various combinations around the six carbon inositol ring. Each of the resulting molecules—inositol phosphates (InsPs)—have a distinct three-dimensional phosphate pattern that can encode unique signalling properties. Within this family of signalling molecules, there is a subgroup that possess functionally significant, ‘high-energy’ diphosphate groups: the inositol pyrophosphates (also known as diphosphoinositol polyphosphates) [1] , [2] . These molecules, particularly InsP 7 and InsP 8 , are now viewed as being of fundamental importance in all eukaryotes [2] . Inositol pyrophosphates play pivotal roles in several aspects of cellular and organismic metabolic homeostasis [1] , [3] , [4] , [5] , [6] , [7] , and they regulate interferon transcription in response to viral infection [8] . Indeed, cell signalling by the inositol pyrophosphates is considered to be among the most evolutionarily ancient functions of the entire inositol phosphate family [9] . Thus, there is considerable interest in the kinases that synthesize InsP 7 and InsP 8 . For example, mammals express three isoforms of inositol hexakisphosphate kinases (IP6Ks) [10] , [11] that each add a second phosphate group to a preexisting phosphate at the 5-position of the inositol ring. These kinases thereby convert InsP 6 to 5-PP-Ins(1,2,3,4,6)P 5 (5-InsP 7 ) [12] , [13] . The type 1 and type 2 isoforms (IP6K1 and IP6K2, respectively) have been the subject of a number of genetic studies with startling phenotypes. Silencing of IP6K1 in pancreatic β-cells inhibits insulin secretion [4] . Gene disruption of murine IP6K1 increases the insulin sensitivity of target tissues [14] , reduces spermatogenesis [14] and compromises haemostasis [15] . Furthermore, in MEFs prepared from IP6K1 −/− mice, DNA repair by homologous recombination is impaired [16] , the epigenetic program is altered [17] and mitochondria are defective [3] . A reduction in IP6K2 expression through an antisense strategy reduces apoptosis [18] , while IP6K2 −/− mice show increased susceptibility to carcinogen-induced squamous cell carcinoma [19] . As IP6Ks have so many important functions, the determination of their structures is a key research goal: such information illuminates catalytic mechanisms, regulatory processes and evolutionary relationships with other kinases, while also offering templates for the rational design of selective inhibitors as research tools or for therapeutic applications. However, IP6Ks have been stubbornly resistant to structural analysis for many years. Our goal has been to fill this significant void in our structural and molecular understanding, so as to further our insight into the entire inositol phosphate kinase family. Entamoeba histolytica express an intriguing IP6K homologue (Genbank: XP_648490.2) that, secondary to its InsP 6 kinase activity, also phosphorylates the 6-OH of Ins(1,4,5)P 3 (ref. 20 )—an inositol phosphate multikinase (IPMK)-like activity [10] , [21] , [22] . IPMK itself is positionally promiscuous in that it is a 3-, 5- and 6-kinase [23] . Another nonspecific inositol phosphate kinase is ITPK1, which phosphorylates the 1-, 5- and 6-positions around the inositol ring [24] . Within the active sites of IPMK and ITPK1, the plane of the inositol rings in all of the alternate substrates are proposed to occupy the same spatial orientation, enabling each substrate to interact with a common set of protein contacts [25] , [26] , [27] , [28] . However, there has not previously been any direct structural confirmation of that hypothesis, because the published crystal structures of IPMK [26] , [28] and ITPK1 [27] , [29] lack bound substrate. We therefore considered that structural analysis of the IP6K from E. histolytica could generate new ideas concerning specificity determinants of the positional promiscuity of inositol phosphate kinases. IP6Ks are members of a wider inositol phosphate kinase family (Pfam PF03770) that includes IPMKs and inositol trisphosphate kinases (IP3Ks); these enzymes all share a PxxxDxKxG (‘PDKG’) catalytic motif [10] , [21] . Phylogenetic analysis [9] has led to the hypothesis that this kinase family arose from a primordial IP6K precursor. However, such an evolutionary pathway would be highly unusual, at least according to current thinking [30] . The issue of concern is that the original substrate (InsP 6 ) for the putative progenitor kinase is both larger and substantially more polar than the substrates for the descendant kinases: the InsP 3 and InsP 4 that are phosphorylated by IPMKs [26] , [28] and the InsP 3 that is specifically phosphorylated at the 3-OH by IP3Ks [31] , [32] . The traditional viewpoint is that improvements in the efficiency of catalysis of the smaller substrates (InsP 3 /InsP 4 ) would evolve through the compression of the active site [30] . However, that would generally be expected to reduce activity against the larger InsP 6 molecule—a ‘negative trade-off’—that would impede organismic fitness and thereby select against the emergence of the independent InsP 3 /InsP 4 kinase activities [30] . Such restrictions would seem inevitable if all substrates interacted with common structural elements. Nevertheless, the significant InsP 3 kinase activity of E. histolytica IP6K [20] suggests it has somewhat overcome the constraints of negative trade-off; structural analysis could reveal how this was accomplished. We now describe several crystal complexes of the IP6K from E. histolytica , including those that contain either large (Ins(1,3,4,5,6)P 5 /InsP 6 ) or small (Ins(1,4,5)P 3 ) substrates. Furthermore, we extrapolate our findings to mammalian IP6Ks by site-directed mutagenesis of the human IP6K2. We describe two structural elements, an α-helical pair and a rare, two-turn 3 10 helix, that together form a substrate-binding pocket with an open clamshell geometry. InsP 6 has substantial contacts with both structural elements. Relative to InsP 6 , enzyme-bound InsP 3 rotates 55° closer to the α-helices, which provide most of the protein’s interactions with InsP 3 . These data provide insight into the molecular determinants of both IP3Ks and IP6Ks, and suggest an unusual evolutionary trajectory for propagation of these separate kinases. Ins(1,4,5)P 3 , InsP 5 and InsP 6 phosphorylation by Eh IP6KA In our study, a recently characterized IP6K expressed by E. histolytica [20] (Genbank: XP_648490.2) is referred to as Eh IP6KA, in order to distinguish it from two other gene products of E. histolytica that are currently also annotated as IP6Ks in Genbank. High-performance liquid chromatography (HPLC) of the InsP 7 synthesized by Eh IP6KA (solid line, Fig. 1a ) found it to co-elute with the 5-InsP 7 produced by Hs IP6K2 (ref. 12) [12] (dotted line, Fig. 1a ). A previous study [20] also concluded from HPLC that Eh IP6KA synthesizes 5-InsP 7 . Nevertheless, current HPLC methodology alone does not completely resolve all possible InsP 7 isomers [33] , [34] . Furthermore, there have been reports that amoeba contain atypical isomers of inositol pyrophosphates [35] . Considering that positional specificity is such a central feature of our study (see the Introduction), we employed nuclear magnetic resonance (NMR) for definitive characterization of the InsP 7 product [12] , [13] . 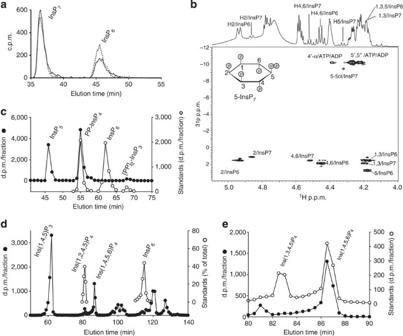Figure 1: HPLC and NMR analysis of the products of Ins(1,4,5)P3and InsP6phosphorylation byEhIP6KA. (a) HPLC analysis (Partisphere SAX, Gradient 1; see Methods) of InsP6phosphorylation by eitherEhIP6KA (57 ng, 20 min; solid line) orHsIP6K2 (7.6 ng, 20 min; dotted line). (b) NMR analysis of the products of the reaction between InsP6and ATP catalysed byEhIP6KA; the figure depicts an overlay of the 1D1H and 2D 1H/31P HSQC spectra. The acquisition parameters are given under Methods. (c) HPLC analysis (Partisphere SAX, Gradient 2; see Methods) of the phosphorylation of ~\n9,000 d.p.m. [14C]Ins(1,3,4,5,6)P5byEhIP6KA (6 μg, 20 min, 50 μl; filled circles). Also shown are the elution of [3H]-labelled internal standards of PP-InsP4and [PP]2-InsP3, as well as InsP6(open circles). (d,e) depict representative HPLC assays (90 min; 200 μl) that contained ~\n10,000 d.p.m. [3H]Ins(1,4,5)P3plus 2 μgEhIP6KA. After quenching and neutralization, products (filled circles) were analysed by Q100 SAX HPLC (Gradient 3);dincludes the elution positions of standards of [3H]Ins(1,2,4,5)P4and [3H]InsP6(open circles), determined in parallel HPLC runs;ezooms in on the InsP4region of the chromatograph; elution of internal [14C] standards of Ins(1,3,4,5)P4and Ins(1,4,5,6)P4are also shown (open circles). Figure 1: HPLC and NMR analysis of the products of Ins(1,4,5)P 3 and InsP 6 phosphorylation by Eh IP6KA. ( a ) HPLC analysis (Partisphere SAX, Gradient 1; see Methods) of InsP 6 phosphorylation by either Eh IP6KA (57 ng, 20 min; solid line) or Hs IP6K2 (7.6 ng, 20 min; dotted line). ( b ) NMR analysis of the products of the reaction between InsP 6 and ATP catalysed by Eh IP6KA; the figure depicts an overlay of the 1D 1 H and 2D 1H/ 31 P HSQC spectra. The acquisition parameters are given under Methods. ( c ) HPLC analysis (Partisphere SAX, Gradient 2; see Methods) of the phosphorylation of ~\n9,000 d.p.m. [ 14 C]Ins(1,3,4,5,6)P 5 by Eh IP6KA (6 μg, 20 min, 50 μl; filled circles). Also shown are the elution of [ 3 H]-labelled internal standards of PP-InsP 4 and [PP] 2 -InsP 3 , as well as InsP 6 (open circles). ( d , e ) depict representative HPLC assays (90 min; 200 μl) that contained ~\n10,000 d.p.m. [ 3 H]Ins(1,4,5)P 3 plus 2 μg Eh IP6KA. After quenching and neutralization, products (filled circles) were analysed by Q100 SAX HPLC (Gradient 3); d includes the elution positions of standards of [ 3 H]Ins(1,2,4,5)P 4 and [ 3 H]InsP 6 (open circles), determined in parallel HPLC runs; e zooms in on the InsP 4 region of the chromatograph; elution of internal [ 14 C] standards of Ins(1,3,4,5)P 4 and Ins(1,4,5,6)P 4 are also shown (open circles). Full size image To prepare sufficient quantities of pure InsP 7 for NMR analysis, we adopted a strategy that has proved useful in the past [12] , namely, to analyse reaction mixtures ( Fig. 1b ). The 1 H chemical shifts of the unreacted InsP 6 and the product InsP 7 were assigned by comparison with reported InsP 6 chemical shifts [13] and from an analysis of the 2D 1 H– 1 H COSY spectrum of the reaction mixture ( Supplementary Table 1 ). The proton resonances from InsP 6 and InsP 7 are labelled in the 1D 1 H spectrum ( Fig. 1b ). The integral from the InsP 6 protons in the 4/6 positions is approximately three times larger than the corresponding integral arising from the PPInsP 5 product, indicating that about 25% of the InsP 6 was phosphorylated. To verify the assignments and differentiate the InsP 6 and InsP 7 resonances, the 1D 1 H and 31 P spectra were reacquired after spiking the sample with an additional 100 μl of 5 mM InsP 6 . The major difference between the InsP 6 and InsP 7 in the new 1 H spectrum is that the resonance from H-5 is shifted to higher chemical shift and no longer overlaps the H-1,3 resonances as it does in InsP 6 (see also Supplementary Table 1 ). The remainder of the 1 H resonances exhibit less dramatic changes relative to the corresponding resonances in InsP 6 . The H-1,3 and H-4,6 resonances of InsP 7 are equivalent due to the symmetry of molecule. These data are consistent with the site of phosphorylation being at the 5-position. With the 1 H chemical shift assignments in hand, the 31 P chemical shifts of InsP 7 were assigned from a combined analysis of 2D 1 H– 31 P HSQC and 31 P– 31 P COSY spectra ( Supplementary Table 1 ). The HSQC spectrum correlates the 1 H shifts at each site to the 31 P shifts of the phosphate on the same carbon, and the COSY spectrum correlates the 31 P shifts of the two 31 P nuclei in the diphosphate moiety. The H-2, H-1,3 and H-4,6 proton chemical shifts correlate to 31 P chemical shifts from the monophosphate groups in InsP 7 , and the H-5 proton shift correlates to the 31 P chemical shift of the α-phosphate of the only diphosphate group ( Fig. 1b ), so we conclude that the site of phosphorylation is the 5-position. Note the two other α-phosphate resonances arise from the ADP product and from unreacted ATP ( Fig. 1b ). The β-phosphate chemical shift of InsP 7 is assigned from its correlation to the α-phosphate chemical shift in the 31 P– 31 P COSY spectrum. Thus, our NMR data reinforce the conclusion reached by HPLC that Eh IP6KA, like mammalian IP6Ks, converts InsP 6 to 5-InsP 7 . Mammalian IP6Ks also phosphorylate Ins(1,3,4,5,6)P 5 , yielding PP-InsP 4 [12] , [36] . We found that Eh IP6KA likewise phosphorylates Ins(1,3,4,5,6)P 5 , and the major product co-elutes with a PP-[ 3 H]InsP 4 standard [12] , [36] ; no InsP 6 was formed ( Fig. 1c ). A small amount of [PP] 2 -InsP 3 [12] , [36] also accumulated ( Fig. 1c ). The first order rate constant for Ins(1,3,4,5,6)P 5 phosphorylation (mean±s.e. ; 0.15±0.006 s −1 mg −1 , n =3) is 40-fold lower than that for InsP 6 (6.1±0.64 s −1 mg −1 , n =3). The rate of phosphorylation of Ins(1,4,5)P 3 , another Eh IP6K substrate [20] , was 0.028±0.005 s −1 mg −1 ( n =3), which is 220-fold slower than that for InsP 6 . HPLC indicates that Ins(1,4,5,6)P 4 is the major InsP 4 product formed from Ins(1,4,5)P 3 ( Fig. 1d,e ) [20] . We also observed the accumulation of an additional InsP 4 isomer that co-elutes with a standard of Ins(1,2,4,5)P 4 ( Fig. 1d ). The phosphorylation of an inositol phosphate at the 2-position has only previously been observed for IP5K [26] , [37] . We also confirmed that there were no pyrophosphorylated molecules associated with the InsP 4 products, because these were not dephosphorylated upon their incubation with DIPP1 ( Supplementary Fig. 1 ), an inositol pyrophosphate phosphatase that removes the β-phosphate from the diphosphate group [36] , [38] . Overall structure of Eh IP6KA The structure of Eh IP6KA ( Fig. 2a–c ; Table 1 ) was determined through two approaches. First, the structure of the fusion protein MBP- Eh IP6KA (apo-enzyme; residues 32–270, space group P2 1 2 1 2 1 ) was determined by a molecular replacement approach using MBP (1ez9) and IP3K (1w2c) as search models. That information was then used for further molecular replacement in order to solve the structures of crystal complexes that bound ATP plus either Ins(1,4,5)P 3 , Ins(1,3,4,5,6)P 5 or InsP 6 (residues 27–270, space group I4 1 22), and a crystal of the apo-enzyme (residues 20–270, space group P2 1 ). In the latter, the amino-terminal residues 20–29 were disordered. 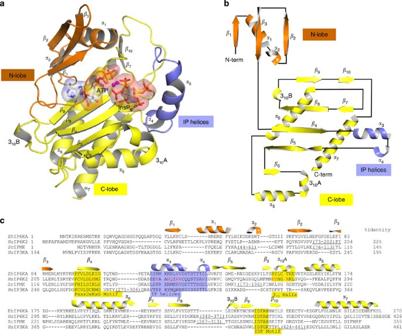Figure 2: Overall structure ofEhIP6KA. (a) Ribbon-plot ofEhIP6KA structure. ATP and InsP6are shown as sticks within a transparent surface. Two Mg atoms are depicted as magenta balls. (b) Topology diagram. (c) A manual alignment of amino-acid sequences (EhIP6KA, XP-648490.2;HsIP6K2, NP_057375.2;ScIPMK, NP_010458.3;HsIP3KA, NP_002211.1), guided by the structural elements that have been observed in crystal structures, and in the case ofHsIP6K2, secondary structural predictions. Outside of the conserved catalytic core of theHsIP6K2 are two significant insertions that are omitted from the alignment. The first of these (residues 73–202) includes a specialized HSP90-binding domain54. The second insertion (residues 340–371) includes a CK2-regulated, ubiquitination motif55. The secondary structural elements fromEhIP6KA are depicted above its sequence and are color-coded orange for the N-lobe, yellow for the C-lobe and blue for the IP helices. Structural elements that directly participate in substrate interactions are highlighted by shading. Residues inHsIP6K2 that were selected for mutagenesis are coloured red. PDB codes forEhIP6KA are 4O4B, 4O4C, 4O4D, 4O4E, 4O4F. Figure 2: Overall structure of Eh IP6KA. ( a ) Ribbon-plot of Eh IP6KA structure. ATP and InsP 6 are shown as sticks within a transparent surface. Two Mg atoms are depicted as magenta balls. ( b ) Topology diagram. ( c ) A manual alignment of amino-acid sequences ( Eh IP6KA, XP-648490.2; Hs IP6K2, NP_057375.2; S cIPMK, NP_010458.3; Hs IP3KA, NP_002211.1), guided by the structural elements that have been observed in crystal structures, and in the case of Hs IP6K2, secondary structural predictions. Outside of the conserved catalytic core of the Hs IP6K2 are two significant insertions that are omitted from the alignment. The first of these (residues 73–202) includes a specialized HSP90-binding domain [54] . The second insertion (residues 340–371) includes a CK2-regulated, ubiquitination motif [55] . The secondary structural elements from Eh IP6KA are depicted above its sequence and are color-coded orange for the N-lobe, yellow for the C-lobe and blue for the IP helices. Structural elements that directly participate in substrate interactions are highlighted by shading. Residues in Hs IP6K2 that were selected for mutagenesis are coloured red. PDB codes for Eh IP6KA are 4O4B, 4O4C, 4O4D, 4O4E, 4O4F. Full size image Table 1 Data collection and structure refinement statistics. Full size table For each asymmetric unit, our data are consistent with one molecule of MBP- Eh IP6KA in space group P2 1 2 1 2 1 , one molecule of substrate-bound Eh IP6KA in space group I4 1 22 and two molecules of apo- Eh IP6KA in space group P2 1 . The latter crystal structure was analysed with the protein interfaces, surfaces and assemblies service ( https://www.ebi.ac.uk/pdbe/pisa/ ), which estimated an interface area of 814.7 Å 2 and total gained free energy upon interface formation of −10.8 kcal mol −1 . It was also assigned a complexation significance score of zero, indicating that the apo structure is a monomer. Furthermore, gel filtration indicates that apo- Eh IP6KA is a monomer in solution. Analysis of the overall fold of Eh IP6KA ( Fig. 2a,b ) offers a description of some architectural elements that are shared with IPMKs and IP3Ks, while also revealing some molecular differences that may contribute to individual catalytic preferences. Among conserved elements, we identified domains in Eh IP6KA that are similar to the so-called N- and C-domains that comprise the ATP-binding sites in both IPMK [26] , [28] and Hs IP3KA [31] , [32] . First, an N-terminal lobe in Eh IP6KA can be designated from residues 28–91, which consist of three antiparallel β-strands; the β1 and β2 strands are connected by two short helices α1 and α2. Second, we can designate a C-terminal lobe (residues 92–102 and 132–270), which is an α+β fold with five, central antiparallel β-strands including β4–6, as well as β8 and β9 (connected by a 3-residue 3 10 helix), a pair of small antiparallel β-strands (β7 and β10), and three α-helices (α5–α7). Also in the C-lobe of Eh IP6KA, between the β6 strand and the α5 helix, is an unusually long (6-residue), two-turn 3 10 helix (3 10 A; Fig. 2a ) that is not present in either IPMK [26] , [28] or Hs IP3KA [31] , [32] . A 3 10 helix of this length occurs relatively rarely because, being thinner and more tightly wound than classical α-helices, it would usually be too unstable [39] , [40] . However, as we describe below, the highly specialized nature and orientation of the amino-acid side chains in this 3 10 helix not only stabilize this structural element, but also make it functionally integral to substrate binding by Eh IP6KA. Description of the nucleotide-binding region of Eh IP6KA We observed that ATP is sandwiched between the N- and C-lobes of Eh IP6KA ( Fig. 2a ); nucleotide binding did not alter protein conformation. Within a conserved IDF tripeptide ( Fig. 2c ) is Asp231, which coordinates with two Mg ions and makes polar contacts with the nucleotide phosphates ( Fig. 3a,b ). The orientation of the nucleotide in Eh IP6KA is superimposable upon its position in the other kinases that share the PDKG motif, except for the more flexible γ-phosphate of ATP ( Fig. 3c ; Supplementary Fig. 2 ), which may contribute to the unusually low affinity of IP6Ks for this nucleotide [41] . The adenosine moiety of ATP is docked in a hydrophobic pocket in Eh IP6KA that is surrounded by residues Leu36, Pro65, Met85, Asn87, Met89 from the N-lobe and Leu211 and Ile230 from the C-lobe ( Figs 3a and 4a ). The N 1 and N 6 atoms of adenine are hydrogen bonded with the amide nitrogen and carbonyl oxygen of Leu88 and Glu86 respectively, which anchors the adenosine in the hydrophobic pocket ( Figs 3a and 4a ). The ATP-ribose group is loosely confined by several Van der Waals contacts with Val97, Asp99, Leu211 and Ile230. Lys38 forms two hydrogen bonds with oxygen atoms from the α- and β-phosphates ( Figs 3a and 4a ). 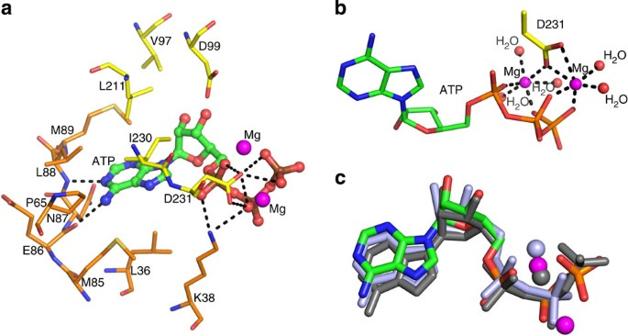Figure 3: Nucleotide binding byEhIP6KA. (a) ATP is depicted as a stick and ball model. Two Mg atoms are depicted as magenta spheres. Polar contacts are shown with dashed lines. Amino acids are shown as stick models. (b) Metal coordination. Two Mg atoms are depicted as magenta spheres. Water molecules are depicted as red spheres. The structure of ATP and Asp231 is shown as stick models. Polar contacts to coordinate with Mg atoms are shown with dashed lines. (c) The orientation of theEhIP6KA-bound nucleotide (green for carbon, red for oxygen, blue for nitrogen and orange for phosphorus atoms) and Mg atoms (magenta spheres) are superimposed upon that forHsIP3KA (grey stick represent AMPPNP (ATP analogue); grey spheres represent Mg), andScIPMK (light blue stick and spheres represent ADP and Mg). Figure 3: Nucleotide binding by Eh IP6KA. ( a ) ATP is depicted as a stick and ball model. Two Mg atoms are depicted as magenta spheres. Polar contacts are shown with dashed lines. Amino acids are shown as stick models. ( b ) Metal coordination. Two Mg atoms are depicted as magenta spheres. Water molecules are depicted as red spheres. The structure of ATP and Asp231 is shown as stick models. Polar contacts to coordinate with Mg atoms are shown with dashed lines. ( c ) The orientation of the Eh IP6KA-bound nucleotide (green for carbon, red for oxygen, blue for nitrogen and orange for phosphorus atoms) and Mg atoms (magenta spheres) are superimposed upon that for Hs IP3KA (grey stick represent AMPPNP (ATP analogue); grey spheres represent Mg), and Sc IPMK (light blue stick and spheres represent ADP and Mg). 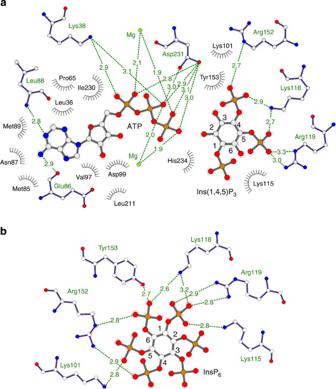Figure 4: Ligplots showing interactions ofEhIP6KA with ATP and InsPs. Ligplots are shown for (a), ATP and Ins(1,4,5)P3and (b), InsP6. Hydrogen bonds are shown in green dashed lines; bond distances are denoted in Angstroms. Residues that make hydrophobic interactions are depicted as grey eyelashes (cutoff distance is 3.9 Å). Atoms are shown white for carbon, red for oxygen, blue for nitrogen and orange for phosphorus. Full size image Figure 4: Ligplots showing interactions of Eh IP6KA with ATP and InsPs. Ligplots are shown for ( a ), ATP and Ins(1,4,5)P 3 and ( b ), InsP 6 . Hydrogen bonds are shown in green dashed lines; bond distances are denoted in Angstroms. Residues that make hydrophobic interactions are depicted as grey eyelashes (cutoff distance is 3.9 Å). Atoms are shown white for carbon, red for oxygen, blue for nitrogen and orange for phosphorus. Full size image The molecular determinants of inositol phosphate binding We have obtained crystal structures of Eh IP6KA in complex with three different substrates: Ins(1,4,5)P 3 , Ins(1,3,4,5,6)P 5 and InsP 6 ( Figs 4a,b and 5a–d , Supplementary Fig. 3 ). Simulated annealing omit-maps and 2 F o− F c maps show clear density of the substrate’s inositol ring; the individual phosphate groups and their specific positions can each be identified ( Supplementary Fig. 3 ). 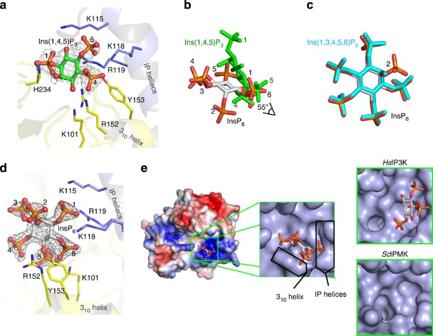Figure 5: Inositol phosphate-binding site forEhIP6KA. (a) Binding of Ins(1,4,5)P3(stick and ball model; green for carbon, red for oxygen and orange for phosphorus atoms. The phosphate groups are numbered). The refined 2Fo−Fcelectron density map is contoured at 1.3σ. (b) Overlay of InsP6(grey stick model with orange and red phosphate groups) and Ins(1,4,5)P3(green stick). (c) Overlay of InsP6and Ins(1,3,4,5,6)P5(cyan stick). (d) Binding of InsP6(stick and ball model; green for carbon, red for oxygen and orange for phosphorus atoms). The phosphate groups are numbered. Amino acids are shown as stick models. The refined 2Fo−Fcelectron density map is contoured at 1.3σ. (e), Electrostatic surface plot with blue and red coloration to respectively indicate positive and negative electrostatic potentials at physiological pH. In the magnified surface representation, the positions of the 310helix and IP helices are highlighted. Bound InsP6is depicted as a stick model. Also shown are surface representation of Ins(1,4,5)P3in the active site ofHsIP3K (data from ref.32) and the active site ofScIPMK (data from ref.26; crystals did not contain substrate). Figure 5: Inositol phosphate-binding site for Eh IP6KA. ( a ) Binding of Ins(1,4,5)P 3 (stick and ball model; green for carbon, red for oxygen and orange for phosphorus atoms. The phosphate groups are numbered). The refined 2 F o − F c electron density map is contoured at 1.3 σ . ( b ) Overlay of InsP 6 (grey stick model with orange and red phosphate groups) and Ins(1,4,5)P 3 (green stick). ( c ) Overlay of InsP 6 and Ins(1,3,4,5,6)P 5 (cyan stick). ( d ) Binding of InsP 6 (stick and ball model; green for carbon, red for oxygen and orange for phosphorus atoms). The phosphate groups are numbered. Amino acids are shown as stick models. The refined 2 F o − F c electron density map is contoured at 1.3 σ . ( e ), Electrostatic surface plot with blue and red coloration to respectively indicate positive and negative electrostatic potentials at physiological pH. In the magnified surface representation, the positions of the 3 10 helix and IP helices are highlighted. Bound InsP 6 is depicted as a stick model. Also shown are surface representation of Ins(1,4,5)P 3 in the active site of Hs IP3K (data from ref. 32 ) and the active site of Sc IPMK (data from ref. 26 ; crystals did not contain substrate). Full size image The binding site for InsP 6 , which lies in a shallow depression in the enzyme’s surface, can be likened to an ‘open clamshell’. One jaw is represented by the IP helices, the other jaw comprises the 3 10 A helix; note that neither H sIP3KA nor IPMK possess an equivalent to the 3 10 A helix ( Fig. 5e ). The IP helices and the 3 10 helix are not directly connected, but they approach within a sufficient proximity of each other to provide a metaphorical ‘hinge’ to the clamshell. Here, the 1- and 6-phosphates of InsP 6 make contacts with Lys115, Lys118 and Arg119 in the α-3/α-4 helical pair ( Figs 4b and 5d ). Nevertheless, the plane of the inositol ring of InsP 6 runs parallel to the contour of the 3 10 A helix ( Fig. 5e ), enabling the 4- and 6-phosphates to interact with Arg152 and Tyr153 ( Figs 4b and 5d ). These contacts appear to be stabilized by cation–pi interactions between Arg152 and Tyr153, which in turn are facilitated by the specific architecture of the 3 10 helix ( Supplementary Fig. 4 ). Ins(1,3,4,5,6)P 5 is also a substrate for EhIP6K ( Fig. 1c,d ). Indeed, Ins(1,3,4,5,6)P 5 and InsP 6 occupy a similar orientation within the active site ( Fig. 5c ), indicating how both can be phosphorylated at the same position. IP6Ks can also phosphorylate 1-InsP 7 (ref. 13 ). Assuming that InsP 6 and 1-InsP 7 also occupy similar orientations within the active site, molecular modelling indicates that the latter’s β-phosphate projects into the bulk phase and should not greatly influence substrate binding. While it is the 5-phosphate group on InsP 6 that is diphosphorylated by Eh IP6KA ( Fig. 1b ), it is either the 2- or the 6-OH of Ins(1,4,5)P 3 that is phosphorylated ( Fig. 1d,e ). Positional promiscuity in other inositol phosphate kinases has been rationalized by proposing alternative substrate-binding modes, in which the plane of the inositol ring occupies the same spatial orientation relative to the active site, enabling each substrate to share the same protein-contact points [25] , [26] , [27] , [28] . This is not the case for Eh IP6KA. Instead, a unique adaptation of Eh IP6KA lies in the nature of its contacts with Ins(1,4,5)P 3 that tilt the plane of the inositol ring by 55° relative to that of InsP 6 ( Fig. 5b ). Thus, near the clamshell hinge, the 5-phosphate of Ins(1,4,5)P 3 somewhat overlaps the space that would be occupied by the 1-phosphate of InsP 6 ( Fig. 5b ). However, at the open end of the clamshell, the 1-phosphate of Ins(1,4,5)P 3 is positioned 7.5 Å away from the location of the 3-phosphate of InsP 6 ( Fig. 5b ). In fact, steric restrictions prevent InsP 6 from occupying the same space as Ins(1,4,5)P 3 in the substrate-binding pocket. The 3 10 helix makes only limited contact with Ins(1,4,5)P 3 : the 4-phosphate has just one hydrogen bond with Arg152 and there are weak Van der Waals interactions with Tyr153 ( Figs 4a , 5a ). Instead, the plane of the inositol ring in Ins(1,4,5)P 3 is tilted closer to the IP helices, which are what this substrate mainly interacts with. Lys118 and Arg119 make contacts with the 4- and 5-phosphates of Ins(1,4,5)P 3 ( Figs 4a and 5a ). The 1-phosphate, 6-hydroxyl and 5-phosphate of Ins(1,4,5)P 3 also have Van der Waals interactions with Lys115 ( Fig. 4a ). The 2-OH of Ins(1,4,5)P 3 is positioned 3.7 Å from the γ-phosphate of ATP ( Supplementary Fig. 5 ), which is close enough to permit an in-line phosphoryl-transfer reaction [42] . Indeed, our HPLC analysis revealed Ins(1,2,4,5)P 4 to be a product of Ins(1,4,5)P 3 phosphorylation ( Fig. 1d,e ). Furthermore, we remodelled the orientation of the inositol ring in enzyme-bound Ins(1,4,5)P 3 , by flipping it 180° across its 1/4 axis, whereupon the 6-OH of Ins(1,4,5)P 3 was then positioned 2.9 Å from the γ-phosphate of ATP ( Supplementary Fig. 5 ). This rationalizes the 6-kinase activity against Ins(1,4,5)P 3 by Eh IP6KA ( Fig. 1d,e ). Thus, Ins(1,4,5)P 3 can be held in the active site of Eh IP6KA in two alternative, productive orientations, yielding either Ins(1,2,4,5)P 4 or Ins(1,4,5,6)P 4 as products. Another interesting observation is that, within the ligand-binding pocket of Eh IP6KA, the orientation of the plane of the inositol ring of Ins(1,4,5)P 3 shows a remarkable degree of spatial conservation with that for Hs IP3KA ( Fig. 5a,e , Supplementary Fig. 5 ); [32] one inositol ring is simply flipped 180° across its 2,3/5,6 axis relative to the other so that, in Hs IP3KA, the 3-OH that is phosphorylated lies 4.6 Å from the γ-phosphate of ATP ( Supplementary Fig. 5 ), which is within the distance that permits an in-line, phospho-transfer reaction [42] . Thus, our data suggest that Eh IP6KA be considered an enzymatic parallel to a ‘living fossil’ that illuminates the potential nature of a primordial InsP 6 /InsP 3 kinase. In this putative protein, the open clamshell topology of the active site provides a partial diversification of specificity determinants for Ins(1,4,5)P 3 and InsP 6 , prior to its propagation into separate enzymes that could specialize in either of the two catalytic activities. We used mutagenesis to pursue this idea (see below). Molecular modelling and mutagenesis of human IP6K2 So as to consolidate our structural work with Eh IP6KA, and also to extrapolate it to mammalian IP6Ks, we turned to Hs IP6K2 as a model for mutagenic studies. Interestingly, we found that Hs IP6K2 harbours a vestigial Ins(1,4,5)P 3 kinase activity, some five orders of magnitude weaker than the InsP 6 activity ( Fig. 6a ). The products of Ins(1,4,5)P 3 phosphorylation are Ins(1,3,4,5)P 4 and Ins(1,4,5,6)P 4 ( Fig. 6b ). Although the Ins(1,4,5)P 3 kinase activity was relatively low, it was sufficient to permit us to pursue the specificity determinants for each substrate. 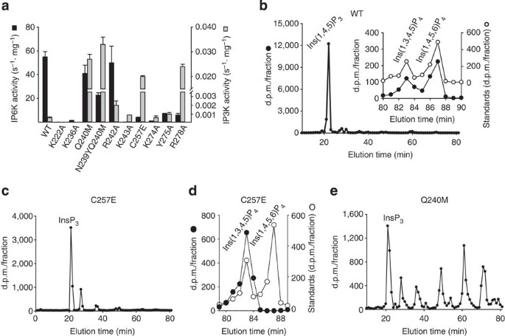Figure 6: HPLC analysis of the kinase activities of wild-type and mutant IP6Ks. (a) InsP6kinase (black bars) and Ins(1,4,5)P3kinase (grey bars) activities of wild-typeHsIP6K2 and the indicated mutants (means±s.e.,n≥3). (b) Shows representative HPLC analysis (Partisphere SAX; Gradient 2) of Ins(1,4,5)P3kinase activities of wild-typeHsIP6K2 (8 μg, 7 h). The inset tobshows HPLC analysis (Q100 SAX; Gradient 3) of the InsP4products formed by the wild-type enzyme (closed circles) together with the elution of internal standards of [14C]-Ins(1,3,4,5)P4and [14C]-Ins(1,4,5,6)P4(open circles). (c) Shows a representative HPLC analysis (Partisphere SAX; Gradient 2) of Ins(1,4,5)P3kinase activity of a Cys257Glu mutant ofHsIP6K2 (5 μg, 1 h). (d) Shows a representative HPLC analysis (Q100 SAX; Gradient 3) of the InsP4products formed by a Cys257Glu mutant ofHsIP6K2 (5 μg, 45 min). (e) Shows a representative HPLC analysis of Ins(1,4,5)P3kinase activity of a Gln240Met mutant ofHsIP6K2 (11 μg, 7 h). WT, wild type. Figure 6: HPLC analysis of the kinase activities of wild-type and mutant IP6Ks. ( a ) InsP 6 kinase (black bars) and Ins(1,4,5)P 3 kinase (grey bars) activities of wild-type Hs IP6K2 and the indicated mutants (means±s.e., n ≥3). ( b ) Shows representative HPLC analysis (Partisphere SAX; Gradient 2) of Ins(1,4,5)P 3 kinase activities of wild-type Hs IP6K2 (8 μg, 7 h). The inset to b shows HPLC analysis (Q100 SAX; Gradient 3) of the InsP 4 products formed by the wild-type enzyme (closed circles) together with the elution of internal standards of [ 14 C]-Ins(1,3,4,5)P 4 and [ 14 C]-Ins(1,4,5,6)P 4 (open circles). ( c ) Shows a representative HPLC analysis (Partisphere SAX; Gradient 2) of Ins(1,4,5)P 3 kinase activity of a Cys257Glu mutant of Hs IP6K2 (5 μg, 1 h). ( d ) Shows a representative HPLC analysis (Q100 SAX; Gradient 3) of the InsP 4 products formed by a Cys257Glu mutant of Hs IP6K2 (5 μg, 45 min). ( e ) Shows a representative HPLC analysis of Ins(1,4,5)P 3 kinase activity of a Gln240Met mutant of Hs IP6K2 (11 μg, 7 h). WT, wild type. Full size image For a positive control in the mutagenic experiments, we prepared a Lys222Ala mutant of Hs IP6K2. This residue (equivalent to Lys101 in Eh IP6KA; Figs 2c , 4b and 5a,d ), lies within the conserved PxxxDxKxG catalytic center ( Fig. 2c ). A Hs IP6K2 construct in which this residue was mutated to Ala has previously been used as a kinase-impaired control when studying the effects of overexpression of wild-type enzyme in intact cells [43] . Nevertheless, to our knowledge, the degree to which this mutation inhibits recombinant enzyme activity has not previously been published. We found that the K222A mutant of Hs IP6K2 exhibits negligible catalytic activity ( Fig. 6a ). Our structural analysis of Eh IP6KA indicates that Lys115 in the IP helices of Eh IP6KA has multiple interactions with both substrates ( Figs 4 and 5 ). We mutated the corresponding Lys236 in Hs IP6K2 ( Fig. 2c ) to Ala; catalytic activity against both substrates was strongly reduced ( Fig. 6a ). Lys118 and Arg119 are two other residues in the IP helices of Eh IP6KA that make contact with both substrates ( Figs 4 and 5 ). These residues are not precisely replicated in Hs IP6K2, according to both our sequence alignments ( Fig. 2c ) and our molecular model of the mammalian kinase ( Supplementary Fig. 6A ). Instead, our modelling indicates that Lys243 in Hs IP6K2 has functionally significant interactions with the 6-phosphate of InsP 6 ( Supplementary Fig. 6A ). Indeed, an Lys243Ala mutation in Hs IP6K2 decreased InsP 6 kinase activity 600-fold ( Fig. 6a ) without affecting Ins(1,4,5)P 3 phosphorylation. These data speak to the specialization of the InsP 6 kinase activity of Hs IP6K2. We next used mutagenesis to test our hypothesis drawn from structural data that the 3 10 A helix in IP6Ks is particularly important for binding InsP 6 . Arg152 and Tyr153 in the 3 10 A helix of Eh IP6KA align with Lys274 and Tyr275 in the equivalent region of Hs IP6K2 ( Fig. 2c ). We found that Lys274Ala and Tyr275Ala mutants of Hs IP6K2 exhibited a decrease in InsP 6 kinase activities of 55- and 8-fold, respectively; the fact that these two mutations did not affect Ins(1,4,5)P 3 kinase activities ( Fig. 6a ) confirms our conclusion that they play only a minor role in binding Ins(1,4,5)P 3 . Interestingly, the 3 10 A helix of Hs IP6K2 contains an Arg residue at position 278 for which there is no equivalent in Eh IP6KA ( Fig. 2c ). Molecular modelling of Hs IP6K2 suggests Arg278 might contribute positive charge to the substrate-binding pocket, and/or stabilize the 3 10 helix through cation–pi interactions with Tyr274 ( Supplementary Fig. 6B ). Consistent with these ideas, an Arg278Ala mutant of Hs IP6K2 exhibited a ninefold reduction in InsP 6 kinase activity compared with wild-type enzyme ( Fig. 6a ). Interestingly, the Arg278Ala mutant also showed a dramatic increase in Ins(1,4,5)P 3 kinase activity ( Fig. 6a ). It is possible Arg278 has a negative impact on Ins(1,4,5)P 3 phosphorylation by attracting it into a nonproductive orientation. The electronegative Glu333 in the C-lobe of Hs IP3KA [32] ( Supplementary Fig. 6C ) is replaced by Ser136 in Eh IP6KA and Cys257 in Hs IP6K2 ( Fig. 2c ). Structural modelling of this region of Hs IP6K2 ( Supplementary Fig. 6B,C ) indicates a Cys257Glu replacement in Hs IP6K2 would cause electrostatic repulsion of InsP 6 but not Ins(1,4,5)P 3 . Indeed, we prepared a Cys257Glu mutant of Hs IP6K2 and it showed 14-fold lower InsP 6 kinase activity than wild-type enzyme ( Fig. 6a ). Moreover, this mutant showed a 33-fold increase in the rate of phosphorylation of Ins(1,4,5)P 3 ( Fig. 6a ), specifically at the 3-OH group ( Fig. 6c,d ). These results indicate the importance of Glu333 in the evolution of catalytic specificity of Hs IP3KA. Finally, a hydrophobic patch in the IP helices in Hs IP3KA and Sc IPMK (Tyr315/Met316 in Hs IP3KA, Met151 in Sc IPMK; Fig. 2c ), against which the inositol ring is proposed to rest, is hypothesized to enhance Ins(1,4,5)P 3 binding [32] . This hydrophobic patch is missing from both Eh IP6KA and Hs IP6K2 ( Fig. 2c ). We introduced Hs IP3KA-like hydrophobic residues into the corresponding region of the IP helices of Hs IP6K2 by preparing a single Gln240Met mutant and a tandem Asn239Tyr/Gln240Met mutant. These two mutant enzymes both exhibited a 50-fold increase in the rate of Ins(1,4,5)P 3 phosphorylation ( Fig. 6a ). Moreover, the variety of products that were formed was significantly increased (compare Fig. 6b and e ), perhaps by favoring multiple ligand-binding modes. Arg242Ala is another mutation that increases the hydrophobicity of the IP helices; this elicited a threefold increase in Ins(1,4,5)P 3 phosphorylation ( Fig. 6a ). Significantly, InsP 6 kinase activity of Hs IP6K2 was not substantially affected by these mutations to Asn239, Gln240 or Arg242 ( Fig. 6a ). These mutagenic data confirm the structural information that indicate InsP 6 and Ins(1,4,5)P 3 have non-overlapping orientations in the substrate-binding site. InsP 6 cannot interact with the synthetic hydrophobic patch since the plane of its inositol ring is tilted away from the plane of the IP helices, unlike that of Ins(1,4,5)P 3 ( Fig. 5b,e ). These mutagenic experiments also offer evolutionary insight by providing proof-of-principle of the nature of mutations to a progenitor kinase that could have increased Ins(1,4,5)P 3 kinase activity without negative trade-off from a compromised InsP 6 kinase activity. In this study, we describe the crystal structure of a bifunctional IP6K/IP3K from E. histoloytica ( Eh IP6KA), and we extrapolate our findings to a human IP6K with mutagenic and biochemical experiments. The most important new ideas that we draw from this information are as follows: first, the geometry of the substrate-binding site is revealed to exhibit a relatively spacious, open clamshell geometry; one jaw is represented by a pair of α-helices, the other jaw is an unusually long 3 10 helix. Second, we show that InsP 3 and InsP 6 have non-overlapping orientations within the substrate pocket. Thus, relatively large InsPs (Ins(1,3,4,5,6)P 5 /InsP 6 ) form contacts with both the α-helices and the 3 10 helix. In contrast, the smaller InsP 3 molecule is rotated 55° closer to the α-helices; the latter provide most of the protein’s interactions with InsP 3 . Third, we describe an unusual evolutionary trajectory that could have favored efficient bifunctionality in a primordial kinase, prior to propagation of separate, dedicated IP3Ks and IP6Ks. Previous ideas concerning how specialized enzymes diverged from promiscuous progenitors are based on the paradigm that the native catalytic activity should generally involve a substrate that is smaller than the emerging substrate, without a change in its degree of polarity [30] . For the putative primordial IP6K [9] , the original, preferred substrate (InsP 6 ) would have been both larger and substantially more polar than the InsP 3 substrates for the emerging kinases (IPMK and IP3K). Usually, the evolution of increased catalytic activity against smaller substrates depends upon compression of the active site [30] . That development would be expected to reduce activity against the larger InsP 6 molecule—a ‘negative trade-off’—that would impede organismic fitness and thereby select against the emergence of the InsP 3 /InsP 4 kinase activities [30] . However, our substrate-bound structures of Eh IP6KA uncover a partial separation of the binding sites for Ins(1,4,5)P 3 and InsP 6 . It is because of these non-overlapping substrate orientations that the insertion of a hydrophobic patch into the α-helices can enhance IP3K activity without affecting IP6K activity: an avoidance of negative trade-off that would have favored efficient bifunctionality. It appears that E. histolytica may be a particularly appropriate model for gaining insight into evolution of a hybrid IP6K/IP3K, since current annotations of this organism’s genome indicate that it does not encode a specialized Ins(1,4,5)P 3 3-kinase. Thus, we conclude that Eh IP6KA is the enzymatic equivalent of a ‘living fossil’ that is suggestive of the nature of a primordial IP6K prior to gene duplication. After the latter event had occurred, it would appear that evolutionary gain of function of Ins(1,4,5)P 3 phosphorylation would then have involved atrophy of the 3 10 helix and consolidation of the role of the IP helices in substrate binding ( Fig. 5e ). In Hs IP3KA, the IP helices have been replaced with a distinct, highly structured 63-residue inositol–phosphate-binding domain: four helices with greater structural constraints that limit substrate selectivity to Ins(1,4,5)P 3 alone [31] , [32] . The 3 10 helix has also been lost from IPMK ( Fig. 5e ), but the substrate-binding pocket remains relatively spacious, thereby retaining a degree of positional promiscuity. Each of the inositol phosphate kinases that share the PDKG motif—IP6Ks, IPMKs and IP3Ks—are specialized to synthesize unique InsPs with differing biological actions. Our molecular understanding of these catalytic specializations has been incomplete, since among these proteins, only Hs IP3KA has previously been co-crystallized with substrate [32] . In contrast, the published crystal structures of IPMK [26] , [28] lacked bound substrate. Thus, our atomic level description of a substrate-bound IP6K fills a significant void in our structural and molecular understanding of the determinants of catalytic activity in the entire PDKG motif kinase family. This information is also relevant to IP5K—previously thought to be the only inositol phosphate kinase capable of phosphorylating the 2-OH. Nevertheless, in crystals of substrate-bound IP5K, the orientation of the axial 2-OH of Ins(1,3,4,5,6)P 5 , relative to ATP, is very similar to the orientation of the equatorial 3-OH of Ins(1,4,5)P 3 , relative to ATP, in crystals of HsIP3KA [44] . Furthermore, the current study shows that the inositol ring of Ins(1,4,5)P 3 occupies very similar relative positions in the active sites of Eh IP6KA and Hs IP3KA ( Fig. 5 ; Supplementary Fig. 5 ). This spatial conservation of substrate binding between these different inositol phosphate kinases is also matched by spatial conservation of some key active-site residues [45] . Such observations help to rationalize our observation that Eh IP6KA phosphorylates Ins(1,4,5)P 3 at the 2-position ( Fig. 1d,e ; Supplementary Fig. 5 ). Finally, our IP6K structure provides the missing template necessary for the rational design of inhibitors that might selectively target each of the different kinases that contain the PDKG motif, both for research tools and therapeutic applications. Protein expression and purification In this study, we use Eh IP6KA as an abbreviation for the E. histolytica IP6K with Genbank accession number XP_648490.2, so as to distinguish it from two other gene products of that are also annotated as IP6Ks. A previous study [20] named this enzyme as Eh IPK1. A codon-optimized cDNA for expression in Escherichia coli of Eh IP6KA was synthesized by Genscript 5′-ATGAACACGAAAATCAAACGCGAACACATGAGTACGAAGAAAAGCCAATGGGTCCAAGCAGGTGGTCACGGTGGTCCGCAACAACTGCATCCGGATGGCCAGTACCTGCTGAAACCGTGCCTGTCCCATCGTGAACGCGACTTTTATCTGCACATTAAAGATGACAAGGAATGGACCGGCACGGGTATTATCCCGAAATTCTACGGCGTCGAACTGCACGAATTTGGCTTCGGTGAACTGGAATTTATCCGTATGGAAAACCTGATGTACAAATACAAGCGCCCGTTCGTTCTGGATCTGAAAATCGGCACCCAAACGTGGGACCCGGAAACCGCGAGCAGCAAAATGAAAAAGCGTCTGGTGGTTGATTCGACCAGCACCACGACCTCTCTGGGCGTGCGTTTTAGTGGTATGGAACGCAATATTGGCGAAGAAAAACCGATCCTGTATTCGCGTTACCTGTGTACCCATGAAGTTAACACGCGCGATAGCCTGAAGGAATACATCAAGCTGTTTTTCAACGACGGTAAAAAGTACCGTAAGGAACTGGTTCCGTACTTTATTAGCCAGCTGGATAAAATGATCGAAGTCATGAAAAAGCGCGAATATAAGATGTTTAGTTCCTCAGTCCTGTTCGTGTACGATTCTACGACCACGCTGGAAGACAAGAAGTACAACTGCAAGATGATCGATTTCGCCCACAATTGGATTCTGTCAGAAGAAGAATGTACCGTGGAAGATGGCTTTCTGTTCGGTCTGAACAATCTGAAATCCATTCTGGAAGACATCGAAAACGAATTTAAGTCACTGTAA-3′. The Gateway Expression System (Invitrogen) was used to subclone Eh IP6KA into the pDest-566 vector. This vector encodes a 6 × His tag, a maltose-binding protein tag and TEV protease cleavage site at the N terminus. ArcticExpress (DE3)-competent cells (Stratagene) were transformed with the resultant plasmid. An overnight culture of E. coli cells carrying the pDest-566- Eh IP6KA was inoculated into 2 × yeast extract tryptone medium at pH 7.5 and grown at 37 °C to A 595 =0.7. Isopropyl β- D -thiogalactopyranoside (0.1 mM) was then added and cultures were continued at 15 °C for 1 day. The cells were disrupted (Constant Systems) at 20 kPsi. Recombinant Eh IP6KA proteins were purified with a Ni-NTA agarose column (Qiagen) followed by a HiTrap Q FF column (GE Healthcare). The bound proteins were released by TEV protease in the presence of 20 mM Tris-HCl (pH 7.5), 50 mM NaCl, 1.5 mM DTT, 10 mM ATP, 20 mM MgCl 2 , then applied to a HiTrap Q FF column. In the case of the MBP fusion protein, this TEV cleavage step was omitted. As a final step, a Superdex 200 gel filtration column (GE Healthcare) was used with a running buffer of 50 mM NaCl and 20 mM Tris-HCl, pH 7.5. Human IP6K2 cDNA was ordered from American Type Culture Collection (I.M.A.G.E. Clone ID 6162048, ATCC number 10437631). The Gateway expression system (Invitrogen) was used to subclone the kinase into the pDest-566 vector. Lemo21(DE3)-competent E. coli cells (New England Biolabs) were transformed with the resultant plasmid. An overnight culture of E. coli cells carrying the pDest-566- Hs IP6K2 was inoculated into 2 × yeast extract tryptone medium supplemented with 0.6 mM L -rhamnose at pH 7.5 and grown at 37 °C to A 595 =0.7. Isopropyl β- D -thiogalactopyranoside (0.1 mM) was then added and cultures were continued at 14 °C for 2 days. The cells were disrupted using a constant cell disruption system (Constant Systems) under 20 kPsi. Recombinant Hs IP6K2 was purified with a Ni-NTA agarose column (Qiagen) followed by a HiTrap Heparin HP column (GE Healthcare), TEV protease cleavage and a HiTrap Q FF column (GE Healthcare). As a final step, a Superdex 200 gel filtration column (GE Healthcare) was used with a running buffer of 150 mM NaCl and 20 mM Tris-HCl, pH 7.5. Mutant proteins were purified similarly. For site-directed mutagenesis, the 5′ version of the complementary primers was as follows (mutagenic nucleotides are emphasized): K222A, 5′-GGTGCCTTGTGTCCTTGACCTC GC GATGGGCACACGACAACATGGTG-3′ K236A, 5′-CAACATGGTGATGATGCTTCAGAGGAG GC GGCAGCCAACCAGATCCGAAAATG-3′ Q240M, 5′-CTTCAGAGGAGAAGGCAGCCAAC ATG ATCCGAAAATGTCAGCAGAGCACATC-3′ N239YQ240M, 5′-GCTTCAGAGGAGAAGGCAGCC T AC ATG ATCCGAAAATGTCAGCAGAGCACATC-3′ R242A, 5′-GGAGAAGGCAGCCAACCAGATC GC AAAATGTCAGCAGAGCACATCTGCAG-3′ K243A, 5′-GAAGGCAGCCAACCAGATCCGA GC ATGTCAGCAGAGCACATCTGCAGTC-3′ K273A, 5′-GTGGGCAGCTCATGTTCATGAAC GC GTACCATGGACGGAAGCTATCGG-3′ Y274A, 5′-GGGCAGCTCATGTTCATGAACAAG GC CCATGGACGGAAGCTATCGGTG-3′ C257E, 5′-GTCATTGGTGTGCGTGTG GAG GGCATGCAGGTGTACCAAG-3′ R278A, 5′-GTTCATGAACAAGTACCATG GA GCGAAGCTATCGGTGCAG-3′ Recombinant DIPP1 was expressed and purified as previously described [46] with an additional, heparin-affinity purification step. The purity of all proteins was estimated to be >95% as judged by SDS–polyacrylamide gel electrophoresis. The purified proteins were concentrated and stored at −80 °C. Sample preparation for NMR analysis Full length Eh IP6KA (1–3 mg) was incubated in 3 ml medium containing 150 mM NaCl, 20 mM Tris-HCl (pH 7.0), 2 mM MgCl 2 , 3 mM ATP and 3 mM InsP 6 at 37 °C for 1 day and then 25 °C for 3 days. The reaction sample was centrifuged and filtered to remove protein, and then vacuum dried at 45 °C for 30 min. The sample was prepared by taking up the reaction mixture in D 2 O to a volume of 600 μl and adjusting the pH to 6.2 using NaOH and HCl. In addition, sodium CDTA was added to a concentration of 20 mM to alleviate broadening of the 31 P resonances due to chemical exchange of the phosphate groups with the high concentration of Mg 2+ in the sample. All 1 H and 31 P chemical shifts were referenced to ~\n5 μM internal DSS or to external 85% phosphoric acid, respectively. All NMR experiments were carried out at 25 °C using a Varian Inova 600 MHz NMR spectrometers, equipped with either a 5 mm broad band NMR probe tuned to 31 P on the observe channel and 1 H on the decoupler channel, or a Varian 5 mm 1 H{ 15 N, 13 C} Cold Probe (Agilent, Santa Clara CA). The 1D 1 H spectra were acquired with sweep widths of 12 p.p.m., with an acquisition time of 1 s, using a 1-s relaxation delay and with presaturation of the residual water resonance during the relaxation delay. The 1D 31 P spectrum was obtained using a 50 p.p.m. sweep width, with an acquisition time of 1.6 s, using a 1-s relaxation delay and with 1 H decoupling during acquisition. The 2D 1 H– 31 P HSQC spectrum was acquired with sweep widths of 12 p.p.m. and 25 p.p.m. in the 1 H and 31 P dimensions, respectively, with 142.3 ms and 42 ms acquisition times in these dimensions and with 1 H decoupling during the acquisition. The 1/4J delay in the HSQC experiment was set to 31.25 ms, corresponding to a 1 H– 31 P scalar coupling of 8 Hz. The 1 H– 1 H and 31 P– 31 P COSY spectra were acquired using gradient-selected absolute value mode COSY experiments. The proton COSY experiment was acquired using 12 p.p.m. sweep widths in both dimensions, with acquisition times of 342 ms and 71 ms in the directly and indirectly detected dimensions, respectively, and with a 1-s relaxation delay, during which time, presaturation of the residual water signal was applied. The phosphorus COSY experiment was acquired using 25 p.p.m. sweep widths in both dimensions, with acquisition times of 512 ms and 32 ms in the directly and indirectly detected dimensions, respectively, and with a 1-s relaxation delay. The 31 P– 31 P COSY spectrum was also acquired with 1 H decoupling in both dimensions. All spectra were processed using Varian VnmrJ 2.2D software (Agilent) on the Varian Inova spectrometer. Enzyme assays and HPLC analysis Kinase assays were performed by incubating enzyme preparations with either [ 3 H]Ins(1,4,5)P 3 (American Radiolabeled Chemicals, Saint Louis, MO), [ 14 C]-Ins(1,3,4,5,6)P 5 (isolated from [ 14 C]-labelled parotid acinar cells [47] ) or [ 3 H]InsP 6 (Perkin-Elmer Waltham MA) at 37 °C in buffer containing 150 mM KCl, 20 mM HEPES pH 7.0, 12 mM MgSO 4 , 10 mM ATP, 1 mM EDTA. After either 20 min (InsP 6 phosphorylation) or 0.5–7 h (Ins(1,4,5)P 3 phosphorylation) reactions were acid quenched and neutralized [48] , and analysed by HPLC using either a 4.6 × 125 mm Partisphere 5 μm SAX column or a Q100 SAX column. The Partisphere column was eluted with one of two ammonium phosphate elution protocols: Gradient 1 (ref. 48) [48] or Gradient 2 (ref. 49) [49] . The Q100 column was eluted with a gradient generated from Buffer A (1 mM Na2EDTA) and Buffer B (Buffer A plus 2 M NH 4 H 2 PO 4 pH 3.9 with H 3 PO 4 ) in the following manner: 0–5 min, 0% B; 5–100 min, 0–42% B, 110–140 min, 42–70% B (Gradient 3). Radioactivity was measured either with an in-line counter, or after collecting 1 ml or 0.5 ml fractions. Other radiolabelled InsPs used for HPLC standards included [ 3 H]Ins(1,2,4,5)P 4 (prepared by heating [ 3 H]Ins(1,3,4,5)P 4 in 0.5 ml 1 M HCl at 90 °C for 20 min [50] ), [ 14 C]-Ins(1,3,4,5)P 4 and [ 14 C]-Ins(1,4,5,6)P 4 (isolated from carbachol-stimulated, [ 14 C]-labelled parotid acinar cells [47] ), PP-[ 3 H]InsP 4 and [PP] 2 -[ 3 H]InsP 3 (both prepared by hIP6K2-mediated phosphorylation of [ 3 H]-Ins(1,3,4,5,6)P 5 [36] ). Data for the kinase assays are presented as mean values±s.e. Crystallization The MBP fusion protein of Eh IP6KA (residues 32–270) was crystallized by hanging drop vapour diffusion against a well buffer of 12% (w/v) PEG 3350, 50 mM NaH 2 PO 4 , pH 5.5 at 18 °C. The protein concentration was >60 mg ml −1 . The core catalytic domain of Eh IP6KA (residues 20–270) was crystallized by hanging drop vapour diffusion for 1 week against a well buffer of 8% (w/v) PEG 3350, 100 mM Na 3 Citrate, pH 5.2 at 25 °C, followed by dilution microseeding (Seed Bead kit, Hampton Research) for 2 weeks with a well buffer of 8% (w/v) PEG 3,350, 100 mM Na 3 Citrate, pH 5.2, 8% ethylene glycol at 25 °C. The crystals were displayed as a thin plate and were anisotropic. Crystals of Eh IP6KA (residues 27–270) emerged under 0.4 M NaH 2 PO 4 in the presence of 10 mM ATP, plus either 10 mM InsP 6 , 5 mM Ins(1,3,4,5,6)P 5 or 5 mM Ins(1,4,5)P 3 /20 mM MgCl 2 . To increase occupancy of InsPs and remove the effect of phosphate ions, the crystals were further soaked under 22% (w/v) PEG 3350, 10 mM MgCl 2 , 10 mM ATP, 0.1 M sodium acetate, pH 5.2 and 20 mM InsP 6 , 10 mM Ins(1,3,4,5,6)P 5 or 10 mM Ins(1,4,5)P 3 for 3 days. Cryosolvent was prepared by adding 33% ethylene glycol into the soaking buffer. Data collection and structure determination Diffraction data were collected using APS beamlines 22-ID and 22-BM. All data were processed with the programme HKL2000 (ref. 51) [51] . Initial phases for the structure of MBP-EhIPK1 were determined by molecular replacement using MBP (1ez9) and Hs IP3KA (1w2c) as searching models. Then the first structure was manually rebuilt with COOT [52] and refined with REFMAC from the CCP4 package [53] . The other crystal structures were determined either by molecular replacement if the space group was different, or by using rigid body and direct Fourier synthesis, and refined with the equivalent and expanded test sets. A Cartesian-simulated annealing protocol was performed in the first round of refinement. Ligand topology and parameter files were prepared using the incorporated PRODRG programme from the CCP4 package [53] . The molecular graphics representations were prepared with the programme PyMol (Schrödinger, LLC). Accession codes : Atomic coordinates and structure factors have been deposited in the Protein Data Bank with accession codes: 4O4B , Eh IP6KA (residues 32–270) tagged with maltose-binding protein at the N terminus; 4O4C , apo- Eh IP6KA (residues 20–270); 4O4D , Eh IP6KA (residues 27–270) in complex with ATP and Ins(1,4,5)P 3 ; 4O4E , Eh IP6KA (residues 27–270) in complex with ATP and Ins(1,3,4,5,6)P 5 ; 4O4F , Eh IP6KA (residues 27–270) in complex with ATP and InsP 6 . How to cite this article : Wang, H. et al. IP6K structure and the molecular determinants of catalytic specificity in an inositol phosphate kinase family. Nat. Commun. 5:4178 doi: 10.1038/ncomms5178 (2014).